ER-localized auxin transporter PIN8 regulates auxin homeostasis and male gametophyte development inArabidopsis Auxin is a key coordinative signal required for many aspects of plant development and its levels are controlled by auxin metabolism and intercellular auxin transport. Here we find that a member of PIN auxin transporter family, PIN8 is expressed in male gametophyte of Arabidopsis thaliana and has a crucial role in pollen development and functionality. Ectopic expression in sporophytic tissues establishes a role of PIN8 in regulating auxin homoeostasis and metabolism. PIN8 co-localizes with PIN5 to the endoplasmic reticulum (ER) where it acts as an auxin transporter. Genetic analyses reveal an antagonistic action of PIN5 and PIN8 in the regulation of intracellular auxin homoeostasis and gametophyte as well as sporophyte development. Our results reveal a role of the auxin transport in male gametophyte development in which the distinct actions of ER-localized PIN transporters regulate cellular auxin homoeostasis and maintain the auxin levels optimal for pollen development and pollen tube growth. The plant hormone auxin has a crucial role in plant development [1] , [2] , [3] , [4] , [5] , [6] . On account of its differential distribution within plant tissues, it acts as a versatile coordinative signal mediating a multitude of processes, including female gametophyte patterning, embryogenesis, organogenesis, meristem activity, growth responses to environmental stimuli and others [7] , [8] , [9] , [10] . High auxin concentration in germinating pollen and active auxin responses in developing pollen [11] , [12] , [13] implicated auxin also in male gametophyte development and function, but its role there remained elusive. A crucial aspect of auxin action is its graded distribution (auxin gradients) that depends on local auxin biosynthesis [14] , [15] , [16] and directional, intercellular auxin transport [7] , [17] , [18] . The polar auxin transport has an essential role in most auxin-regulated processes and is mediated by auxin influx proteins from the AUX1/LAX family [19] , by PIN auxin efflux proteins [20] and by homologues of the ABCB multiple drug resistance transporters [21] , [22] . These auxin transporters typically localize to the plasma membrane (PM) and facilitate auxin flow across the membrane in and out of the cell [23] . Recently, the Arabidopsis thaliana PIN5 auxin transporter has been shown to localize to the endoplasmic reticulum (ER) and its activity is important for the regulation of auxin metabolism [24] . These findings suggest the existence of auxin transport across the ER membrane, although a demonstration of such transport has not been provided yet and its role in auxin biology and plant development is still largely unclear. Here we identify and functionally characterize PIN8, an auxin transporter preferentially expressed in male gametophyte. PIN8 transports auxin across the ER membrane and antagonistically to PIN5 regulates intracellular auxin homoeostasis and metabolism for male gametophyte function. PIN8 is expressed and functions in the male gametophyte To assess a potential role for the auxin transport in male gametophyte development, we examined the expression patterns of PIN auxin transporters by using available transcriptome data [25] . Among the eight members of the PIN protein family in the Arabidopsis genome, a so-far uncharacterized member PIN8 was the only one predominantly expressed in pollen ( Supplementary Fig. S1a ). Reverse transcription PCR confirmed the highly enriched expression of PIN8 in reproductive tissues ( Supplementary Fig. S1b ) and lines comprising the PIN8 coding region fused with green fluorescent protein (GFP) under the control of its native promoter ( PIN8::PIN8-GFP ) showed strong signal in developing and germinating pollen ( Supplementary Fig. S1a ). To analyse the potential role of PIN8 in pollen development, we isolated two insertion mutant alleles, pin8-1 and pin8-2 , disrupting the first and fifth exon of the PIN8 gene, respectively ( Supplementary Fig. S1c,d ). No obvious phenotypic defects were observed in seedlings and adult plants in both alleles (data not shown), which was consistent with very low PIN8 expression in most sporophytic tissues. However, pin8 mutants showed a decreased transmission ability through male gametophyte (38%) for pin8-1 versus the expected 50% for the wild-type (Col-0) pollen ( Fig. 1a ). The complementation of this phenotype confirmed that the described pollen transmission defects are due to the loss of PIN8 function ( Supplementary Fig. S2 ). 4',6-Diamidino-2-phenylindole (DAPI) staining of pollen revealed a high frequency of aborted and misshaped pollen grains in pin8 ( Fig. 1b,c , Supplementary Table S1 ) and transmission electron microscopy analyses showed that pin8 mutant pollen has a reduced density of rough ER (10–15%, n >150 pollen grains) in comparison to the wild-type pollen ( Fig. 1d,e ). Next, we examined transgenic lines overexpressing PIN8 under strong pollen-specific promoter LAT52 (ref. 24 ). LAT52::PIN8 also showed strongly reduced transmission through the male gametophyte (below 10% for LAT52::PIN8 versus expected 50% for the wild-type control; Fig. 1a and Supplementary Fig. S1e ). In addition, in vitro pollen germination assays revealed a decreased pollen germination in pin8 (40% decrease, Fig. 1f ) and increased pollen tube elongation in LAT52::PIN8 lines (30% increase, Fig. 1g ) with a normal pollen tube morphology ( Supplementary Fig. S1f ). Thus, the loss-of-function and ectopic expression analyses revealed a specific role of PIN8 in male gametophyte development and function. 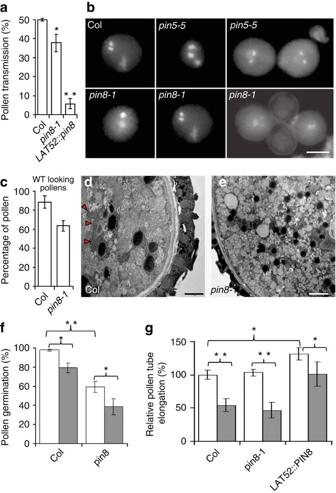Figure 1: PIN8 is involved predominantly in the male gametophyte development. (a) Thepin8mutant and theLAT52::PIN8line showed reduced pollen transmission ability. Error bars represent the standard error of more than ten independent crosses (Student'st-test, *P<0.05). (b,c) DAPI staining analysis showing defects in the morphology ofpin8andpin5mutant pollen. Both mutants showed distorted and/or misplaced male germ unit and less frequently also exhibit pollen mitosis defects. Sometimes, collapsed pollen grains were observed. Scale bar, 10 μm. Error bars represent the standard error of more than 23 independent plants (Student'st-test, **P<0.01). (d,e) Typical ER clusters in wild-type (WT) pollen (d) were not observed in 10–15%pin8pollen (observed 150 pollen grains) (e) by transmission electron microscope analysis. Scale bar, 10 μm. Red arrows mark ER clusters. (f)pin8(2256 pollen were analysed) shows reducedin vitropollen germination abilities (2,814 Col pollens were analysed as the control) and increased sensitivity to auxin treatment (100 nM NAA) with a 35% reduction of pollen germination inpin8(5,017 pollens were analysed) compared with the 19% reduction in Col (1,131 pollens were analysed). Error bars represent the standard error of more than ten independent plants (Student'st-test, *P<0.05; **P<0.01). White and grey columns represent without and with NAA treatment, respectively. (g) Overexpression ofPIN8in pollen in theLAT52::PIN8line strongly increased the resistance (with a 24% inhibition of pollen tube length compared with the 46% inhibition in Col) ofin vitropollen germination to NPA (100 μM NPA) treatment. Error bars represent the standard error of more than six independent plants (Student'st-test, *P<0.05; **P<0.01). White and grey column represent without and with NPA treatment, respectively, in Col,pin8orLAT52::PIN8. Figure 1: PIN8 is involved predominantly in the male gametophyte development. ( a ) The pin8 mutant and the LAT52::PIN8 line showed reduced pollen transmission ability. Error bars represent the standard error of more than ten independent crosses (Student's t -test, * P <0.05). ( b , c ) DAPI staining analysis showing defects in the morphology of pin8 and pin5 mutant pollen. Both mutants showed distorted and/or misplaced male germ unit and less frequently also exhibit pollen mitosis defects. Sometimes, collapsed pollen grains were observed. Scale bar, 10 μm. Error bars represent the standard error of more than 23 independent plants (Student's t -test, ** P <0.01). ( d , e ) Typical ER clusters in wild-type (WT) pollen ( d ) were not observed in 10–15% pin8 pollen (observed 150 pollen grains) ( e ) by transmission electron microscope analysis. Scale bar, 10 μm. Red arrows mark ER clusters. ( f ) pin8 (2256 pollen were analysed) shows reduced in vitro pollen germination abilities (2,814 Col pollens were analysed as the control) and increased sensitivity to auxin treatment (100 nM NAA) with a 35% reduction of pollen germination in pin8 (5,017 pollens were analysed) compared with the 19% reduction in Col (1,131 pollens were analysed). Error bars represent the standard error of more than ten independent plants (Student's t -test, * P <0.05; ** P <0.01). White and grey columns represent without and with NAA treatment, respectively. ( g ) Overexpression of PIN8 in pollen in the LAT52::PIN8 line strongly increased the resistance (with a 24% inhibition of pollen tube length compared with the 46% inhibition in Col) of in vitro pollen germination to NPA (100 μM NPA) treatment. Error bars represent the standard error of more than six independent plants (Student's t -test, * P <0.05; ** P <0.01). White and grey column represent without and with NPA treatment, respectively, in Col, pin8 or LAT52::PIN8 . Full size image As PIN8 is a member of the auxin transporter family, it is presumably involved in auxin transport. However, a role of auxin transport in male gametophyte development and function is far from being clear. To address this issue, we pharmacologically manipulated auxin levels and auxin transport during pollen germination and pollen tube growth. Auxin treatments (100 nM α-naphthaleneacetic acid (NAA)) reduced the pollen germination rate in wild type (19% reduction) and pin8-1 pollen showed increased sensitivity to such auxin treatment (35% reduction) ( Fig. 1f ). Furthermore, the auxin transport inhibitor 1- N -naphthylphthalamic acid (NPA) strongly inhibited pollen tube growth and, notably, LAT52::PIN8 pollen showed increased resistance to this NPA effect ( Fig. 1g ). The inhibition of the in vitro pollen tube growth by NPA was apparent only at high concentrations (100 μM) indicating that it might occur through APM1-regulated functions of PIN and ABCB auxin transport proteins, as APM1 is the target at high concentrations of NPA treatment [26] , [27] . The change in sensitivity in pollen tubes overexpressing auxin transport-related protein PIN8 suggests that it is auxin transport-related effect of NPA that affects pollen tube growth. Collectively, these findings hint at an important role of auxin and auxin transport for male gametophyte function and identified the pollen-specific putative auxin transporter PIN8 as an important factor regulating these processes. PIN8 overexpression affects many aspects of plant growth and development To further characterize the function of PIN8, we generated lines overexpressing PIN8 in sporophytic tissues under the control of the strong cauliflower mosaic virus 35S promoter ( PIN8OX ). PIN8OX lines flowered much earlier than wild-type plants ( Fig. 2a,b ), showed enhanced leaf margin serration, especially under short-day growth conditions ( Fig. 2c ) and had much longer hypocotyls than the control ( Fig. 2d,e ), which can be attributed to the increased cell elongation (Fig. 2f and Supplementary Table S2 ). All these plant growth and development phenotypes in PIN8OX suggest a capacity of PIN8 to influence different aspects of plant development, preferentially those where auxin is involved. 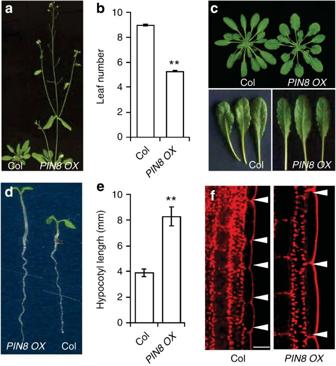Figure 2:PIN8OXlines showed defects in many aspects of plant growth and development. (a,b)PIN8OXlines flower earlier than the wild-type controls measured under long-day growth conditions. Error bars represent the standard error of the mean from three independent experiments (n=48, Student'st-test, **P<0.01). (c)PIN8OXlines showed strongly enhanced leaf margin serration under short-day growth conditions. (d,e)PIN8OXlines showed long hypocotyls compared with the control. Hypocotyl length was measured with 5-day-old seedlings grown under short days. Error bars represent the standard error of the mean from three independent experiments (n=30, Student'st-test, **P<0.01). (f) The cell length inPIN8OXlines is more than two times longer than that in the control (see the quantification data inSupplementary Table S2). The arrows indicate the intercellular space. Scale bar, 10 μm. Figure 2: PIN8OX lines showed defects in many aspects of plant growth and development. ( a , b ) PIN8OX lines flower earlier than the wild-type controls measured under long-day growth conditions. Error bars represent the standard error of the mean from three independent experiments ( n =48, Student's t -test, ** P <0.01). ( c ) PIN8OX lines showed strongly enhanced leaf margin serration under short-day growth conditions. ( d , e ) PIN8OX lines showed long hypocotyls compared with the control. Hypocotyl length was measured with 5-day-old seedlings grown under short days. Error bars represent the standard error of the mean from three independent experiments ( n =30, Student's t -test, ** P <0.01). ( f ) The cell length in PIN8OX lines is more than two times longer than that in the control (see the quantification data in Supplementary Table S2 ). The arrows indicate the intercellular space. Scale bar, 10 μm. Full size image PIN8 and PIN5 localize to the ER In Arabidopsis , the PIN auxin transporter family can be divided in two subclades: one represented by PIN1, PIN2, PIN3, PIN4 and PIN7, which all localize to the PM [23] , and the other subclade represented by PIN5, PIN8 and possibly PIN6, which are characterized by a reduced middle hydrophilic loop [23] and for which PIN5 has been shown to localize to the ER in Arabidopsis [24] . To investigate the subcellular localization of PIN8, we examined Arabidopsis transgenic lines expressing a functional PIN8::PIN8-GFP construct. In PIN8::PIN8-GFP ( Supplementary Fig. S2) , a specific intracellular signal was observed only in pollen and growing pollen tubes ( Fig. 3a–c and Supplementary Fig. S1a ) consistent with the PIN8 expression data ( Supplementary Fig. S1a ). The PIN8-GFP -expressing cells showed intracellular signals, but no localization to the PM ( Fig. 3a–c ). A pronounced co-localization with the ER-tracer dye [24] suggested the association of PIN8-GFP with the ER ( Fig. 3a–c ). 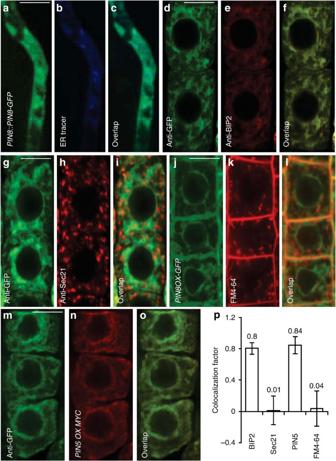Figure 3: PIN8 localizes to the ER. (a–c) PIN8 localization in the pollen tube ofPIN8::PIN8-GFPline and co-localization of PIN8-GFP (green) with the ER-tracker dye (blue). (d–f) PIN8 localization in the root of35S::PIN8-GFPline and co-localization of PIN8-GFP (green) with ER marker BIP2 staining (red). (g–i) PIN8-GFP (green) does not co-localize with Golgi apparatus (GA) marker Sec21 (red). (j–l) PIN8-GFP (green) does not co-localize with endosomes stained with FM4-64 traced (red). (m–o) PIN8-GFP (green) and PIN5-myc (red) co-localize at the ER. (p) The quantification of PIN8 co-localization with ER (anti-BIP2), GA (anti-Sec21), PIN5 (anti-myc) and endosome (FM4-64 staining) markers confirms localization of PIN8 to the ER but not to the GA, endosomes or plasma membrane. The co-localization factor (the highest is 1.0) was calculated by Zeiss software. For microscope observation, 3-day-old seedlings (n=6) and at least five areas were analysed for each seedling. Scale bar, 5 μm. Error bars represent the standard error. Live cell imaging (a–c,j–l) and immunostainings (d–f,g–i,m–o). Figure 3: PIN8 localizes to the ER. ( a – c ) PIN8 localization in the pollen tube of PIN8::PIN8-GFP line and co-localization of PIN8-GFP (green) with the ER-tracker dye (blue). ( d – f ) PIN8 localization in the root of 35S::PIN8-GFP line and co-localization of PIN8-GFP (green) with ER marker BIP2 staining (red). ( g – i ) PIN8-GFP (green) does not co-localize with Golgi apparatus (GA) marker Sec21 (red). ( j – l ) PIN8-GFP (green) does not co-localize with endosomes stained with FM4-64 traced (red). ( m – o ) PIN8-GFP (green) and PIN5-myc (red) co-localize at the ER. ( p ) The quantification of PIN8 co-localization with ER (anti-BIP2), GA (anti-Sec21), PIN5 (anti-myc) and endosome (FM4-64 staining) markers confirms localization of PIN8 to the ER but not to the GA, endosomes or plasma membrane. The co-localization factor (the highest is 1.0) was calculated by Zeiss software. For microscope observation, 3-day-old seedlings ( n =6) and at least five areas were analysed for each seedling. Scale bar, 5 μm. Error bars represent the standard error. Live cell imaging ( a – c , j – l ) and immunostainings ( d – f , g – i , m – o ). Full size image To examine the PIN8 localization in more detail and in different sporophytic cell types, we ectopically expressed PIN8 fused with GFP under the control of 35S promoter. Similar to what was observed in pollen, we detected a consistent, intracellular PIN8-GFP signal co-localized with ER markers, such as BIP2 (ref. 28 ) in root cells ( Fig. 3d–f , p). On the other hand, we did not observe any co-localization of PIN8 with endosomes or Golgi apparatus ( Fig. 3g–i, p and Supplementary Fig. S3 ) and also we did not observe any co-localization with labelled PM ( Fig. 3j–l, p ). Furthermore, PIN8 co-localized with PIN5 at the ER ( Fig. 3m–p ) and this localization was, similar to that of PIN5 (ref. 24 ), insensitive to the treatment with the vesicle trafficking inhibitor brefeldin A ( Supplementary Fig. S4 ). These results strongly suggest that PIN8, similar to PIN5, localizes to the ER and that these proteins might have related functions. PIN8 transports auxin and regulates cellular auxin homoeostasis The ER-localized PIN5 was found, in contrast to PM-localized PIN proteins, not to act in intercellular auxin transport, but to be involved in regulating cellular auxin homoeostasis, presumably by compartmentalizing auxin between the ER and the cytosol [24] . Therefore, we tested the role of PIN8 in regulating auxin homoeostasis. The visualization of auxin responses with the auxin-responsive reporter DR5::GUS [29] revealed no changes in pin8 mutants (data not shown), consistent with a very low expression of PIN8 in sporophytic tissues. In contrast, PIN8OX lines showed a markedly increased DR5 activity, both in the root and in the aerial parts of the seedling ( Fig. 4a ) suggesting elevated auxin levels. 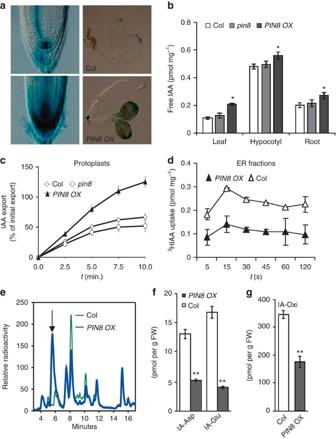Figure 4: PIN8 regulates cellular auxin homoeostasis and auxin transport. (a)PIN8OXexhibits enhanced auxin response as shown by the increasedDR5::GUSactivity in the root and in the aerial parts of the seedling. (b) Changes in free IAA levels inPIN8OXin young leaves/cotyledons, hypocotyls and root tips. Error bars represent the standard error of the mean,n=5 (Student'st-test, *P<0.05). (c) Protoplasts ofPIN8OXshowed a higher rate of IAA export. Error bars represent the standard error of the mean,n=3. (d)3H-IAA uptake time course in ER-enriched membrane fractions from Col andPIN8OXplants. Transport assays were performed as described in Methods. ER-enriched membranes were incubated in 50 nM3H-IAA fractions. Aliquots were taken at different times, filtered and washed. The radioactivity present in the filters was estimated by liquid scintillation counting and expressed as pmol of3H-IAA/mg of total proteins. The experiment was performed two biological repeats, and the error bars represent the standard error of the mean. (e) The HPLC chromatogram of IAA metabolic profile changes noticeably in thePIN8OXline compared with the wild-type control (2.5-h incubation with3H-IAA). (f,g) Liquid chromatography/mass spectrometry detected strongly decreased levels of IAA conjugates (indole-3-acetyl-aspartate, IA–Asp; indole-3-acetyl-glutamate, IA–Glu) (f), and oxindole-3-acetic acid (IA-Oxi) (g) inPIN8OXline. White and grey column represent Col andPIN8OX, respectively. Error bars represent the standard error of the mean,n=3 (Student'st-test, **P<0.01). FW, fresh weigh. Figure 4: PIN8 regulates cellular auxin homoeostasis and auxin transport. ( a ) PIN8OX exhibits enhanced auxin response as shown by the increased DR5::GUS activity in the root and in the aerial parts of the seedling. ( b ) Changes in free IAA levels in PIN8OX in young leaves/cotyledons, hypocotyls and root tips. Error bars represent the standard error of the mean, n =5 (Student's t -test, * P <0.05). ( c ) Protoplasts of PIN8OX showed a higher rate of IAA export. Error bars represent the standard error of the mean, n =3. ( d ) 3 H-IAA uptake time course in ER-enriched membrane fractions from Col and PIN8OX plants. Transport assays were performed as described in Methods. ER-enriched membranes were incubated in 50 nM 3 H-IAA fractions. Aliquots were taken at different times, filtered and washed. The radioactivity present in the filters was estimated by liquid scintillation counting and expressed as pmol of 3 H-IAA/mg of total proteins. The experiment was performed two biological repeats, and the error bars represent the standard error of the mean. ( e ) The HPLC chromatogram of IAA metabolic profile changes noticeably in the PIN8OX line compared with the wild-type control (2.5-h incubation with 3 H-IAA). ( f , g ) Liquid chromatography/mass spectrometry detected strongly decreased levels of IAA conjugates (indole-3-acetyl-aspartate, IA–Asp; indole-3-acetyl-glutamate, IA–Glu) ( f ), and oxindole-3-acetic acid (IA-Oxi) ( g ) in PIN8OX line. White and grey column represent Col and PIN8OX , respectively. Error bars represent the standard error of the mean, n =3 (Student's t -test, ** P <0.01). FW, fresh weigh. Full size image To directly test the role of PIN8 in regulating auxin levels, we measured free auxin (indole-3-acetic acid (IAA)) levels in the pin8 mutant and PIN8OX lines. Unfortunately, free IAA measurements directly in pollen were technically impossible, therefore, we used extraction and gas chromatography/mass spectroscopy detection of IAA in root tips, hypocotyls and rosette leaves. These measurements revealed that loss-of-function pin8 mutants had similar levels of free auxin as the control ( Fig. 4b ), whereas PIN8OX lines showed strongly increased free IAA levels in root tips, hypocotyls and rosette leaves ( Fig. 4b ). Thus, both DR5-monitored auxin response and direct auxin measurements revealed overall elevated auxin levels in plants overexpressing PIN8 . Next, we quantified the auxin efflux from mesophyll protoplasts isolated from rosette leaves of PIN8 loss-of-function and overexpression lines. Consistent with the changes in auxin levels and PIN8 expression data, protoplasts prepared from pin8 mutants exhibited a comparable IAA and NAA efflux as wild-type controls, whereas in protoplasts isolated from PIN8OX , the efflux of IAA and NAA was increased ( Fig. 4c and Supplementary Fig. S5 ), suggesting the auxin transport competence of PIN8. The ER localization of PIN8 in protoplasts ( Supplementary Fig. S6 ) is also consistent with a notion that PIN8 increases efflux of auxin from the ER into the cytoplasm and then presumably out of the protoplast. To directly assess the ability of PIN8 at the ER membranes, we grew PIN8OX -etiolated plants in liquid culture and ER-enriched membrane fractions were prepared using sucrose gradient centrifugation as described [30] . This fraction was well separated from non-ER fractions including Golgi membranes and other organelles. PIN8-GFP was detected in the ER-enriched fraction with an anti-GFP antibody, but no PIN1 was detected with anti-PIN1 (not shown) confirming no or very low PM contamination. Transport assays with radiolabelled IAA showed increased auxin accumulation capacity of the ER fractions from the PIN8OX lines as compared with the control ( Fig. 4d ). In addition, competitive uptake assays with ER-enriched fraction from PIN8OX revealed that synthetic auxins NAA,2,4-D and auxin analogue indole-3-butyric acid can compete with radiolabelled IAA uptake, whereas the biologically inactive analogue benzoic acid (1 mM) did not compete with PIN8-mediated uptake of radiolabelled IAA ( Supplementary Fig. S7a ). Our auxin transport assays in mesophyll protoplasts from transiently transfected nicotiana benthamiana also indicated that IAA, not benzoic acid, was the preferred substrate of PIN8 action ( Supplementary Fig. S7b ). These results show that IAA and other biologically active auxins are preferred substrates of PIN8 action. In an independent set of experiments, lighter ER membranes from PIN8OX seedlings, exhibited acidification after addition of ATP and accumulation of 3 H-IAA in short-term (60 s) uptake assays, whereas denser ER vesicles, tonoplast vesicles and PM vesicles did not show auxin transport activity ( Supplementary Fig. S8 ). The overall increase in auxin responses and free auxin levels in PIN8OX as well as changed auxin transport capacity of PIN8OX protoplasts and ER-derived membranes altogether suggested that PIN8 is an ER-localized auxin transporter involving in the regulation of auxin homoeostasis. To assess the role of PIN8 in IAA metabolism, we analysed the IAA metabolic profile of PIN8OX transgenic seedlings through high-performance liquid chromatography (HPLC). PIN8 overexpression remodelled the IAA metabolism as demonstrated by the pronounced changes in the HPLC profile ( Fig. 4e ). Direct analysis by ultra-high-performance liquid chromatography coupled to tandem mass detection of the selected IAA conjugates confirmed the changes in the IAA metabolic profile and showed that the PIN8OX line had a decreased capacity to produce amino-acid conjugates, such as IA-Asp (indole-3-acetyl-aspartate), IA-Glu (indole-3-acetyl-glutamate) or IA-Oxi (oxindole-3-acetic acid; Fig. 4f,g ). These results demonstrated that the ER-localized PIN8 auxin transporter, similar to PIN5, is also involved in the regulation of auxin homoeostasis. PIN8 and PIN5 act antagonistically To gain additional insights into the roles of PIN5 and PIN8, we systematically compared the loss-of-function and overexpression lines and also generated the pin5 pin8 double mutants and the PIN8OX PIN5OX double transgenic plants. Similar to pin8 , pin5 was also defective in pollen morphology ( Figs 1b , 5a ), but, in contrast to the single pin5 mutant, the pin5 pin8 double mutant largely rescued the pollen morphology defects and the pin8 defect in transmission through the male gametophyte ( Fig. 5a,b ). Thus, the pin5 and pin8 loss-of-function mutants compensated to a large extent each other in male gametophyte development and function. 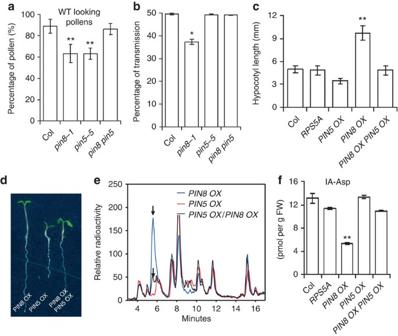Figure 5: PIN8 and PIN5 act antagonistically. (a) Morphological defects in pollen ofpin5(2,400) andpin8(2,400) single mutants were rescued inpin5 pin8(3,300) double mutants as shown by DAPI staining. A total of 7,100 wild-type (WT) pollens were counted as the control. Error bars represent the standard error of more than 23 independent plants (Student'st-test, **P<0.01). (b) The reduced pollen transmission ability in thepin8mutant was rescued in thepin5 pin8double mutant. Error bars represent the standard error of more than ten independent crosses (Student'st-test, *P<0.5). (c,d) The long hypocotyl phenotype of thePIN8OXline was rescued in thePIN8OX PIN5OXline. Error bars represent the standard error of three independent experiments (n=60, Student'st-test, **P<0.01). (e) Specific HPLC chromatogram of IAA metabolic profile ofPIN8OXwas largely rescued in thePIN8OX PIN5OXline (2.5-h incubation with3H-IAA). Arrows indicate the notable changes in the IAA metabolic profile. (f) The decreased free IAA-Asp of thePIN8OXline was rescued in thePIN8OX PIN5OXline. Error bars represent the standard error of the mean,n=3 (Student'st-test, *P<0.05). Figure 5: PIN8 and PIN5 act antagonistically. ( a ) Morphological defects in pollen of pin5 (2,400) and pin8 (2,400) single mutants were rescued in pin5 pin8 (3,300) double mutants as shown by DAPI staining. A total of 7,100 wild-type (WT) pollens were counted as the control. Error bars represent the standard error of more than 23 independent plants (Student's t -test, ** P <0.01). ( b ) The reduced pollen transmission ability in the pin8 mutant was rescued in the pin5 pin8 double mutant. Error bars represent the standard error of more than ten independent crosses (Student's t -test, * P <0.5). ( c , d ) The long hypocotyl phenotype of the PIN8OX line was rescued in the PIN8OX PIN5OX line. Error bars represent the standard error of three independent experiments ( n =60, Student's t -test, ** P <0.01). ( e ) Specific HPLC chromatogram of IAA metabolic profile of PIN8OX was largely rescued in the PIN8OX PIN5OX line (2.5-h incubation with 3 H-IAA). Arrows indicate the notable changes in the IAA metabolic profile. ( f ) The decreased free IAA-Asp of the PIN8OX line was rescued in the PIN8OX PIN5OX line. Error bars represent the standard error of the mean, n =3 (Student's t -test, * P <0.05). Full size image Regarding the overexpression lines, PIN5OX seedlings had shorter hypocotyls [24] , whereas PIN8OX seedlings had strikingly longer hypocotyls than the wild-type control ( Fig. 5c,d ). These overexpression effects were also rescued in the PIN8OX PIN5OX double overexpressing line ( Fig. 5c,d ). In addition, we also observed that pin5 significantly enhanced the long hypocotyl phenotype of PIN8OX further supporting the antagonistic roles of PIN5 and PIN8. ( Supplementary Fig. S9a ). The same could be observed for the flowering time. Under long-day conditions, PIN8OX plants flowered earlier than the control, whereas PIN5OX plants flowered significantly later ( Supplementary Fig. S9b,c ) and the PIN8OX PIN5OX plants flowered at a time that was comparable to the control plants ( Supplementary Fig. S9b,c ). These different observations are also consistent with previous observations on the opposite action of PIN5 and PIN8 in root hair development [31] . Thus, both the loss-of-function mutants and overexpression lines of PIN5 and PIN8 can largely compensate each other in regulating different developmental processes, suggesting antagonistic roles of these two ER-localized PIN proteins. Next, we tested genetic interaction between PIN5 and PIN8 in regulating auxin homoeostasis. In the PIN8OX line, both free IAA measurements and enhanced DR5::GUS activity consistently suggested increased free IAA levels ( Fig. 4 ), whereas PIN5OX had been shown to have decreased auxin levels [24] . To test the possible antagonistic roles of PIN5 and PIN8 in the regulation of auxin metabolism, we measured free IAA levels in PIN8OX PIN5OX double transformants. This analysis revealed that, similar to morphological phenotypes, the increased free IAA levels in PIN8OX were largely rescued in the PIN8OX PIN5OX line that exhibited free IAA levels comparable to those of the control lines ( Supplementary Fig. S10a ). The increased IAA export in protoplasts prepared from PIN8 OX also phenocopies pin5 mutant ( Supplementary Fig. S10b ). Moreover, notable changes in the IAA metabolic profile of PIN8OX seedlings as demonstrated by the HPLC spectrum were also largely rescued in PIN8OX PIN5OX lines ( Fig. 5e ). Accordingly, liquid chromatography–tandem mass spectroscopeanalysis confirmed that the decreased capacity of PIN8OX seedlings to conjugate IAA to amino acids was rescued in the PIN8OX PIN5OX lines ( Fig. 5f ). Overall, the opposite and mutual compensatory effects of pin5 and pin8 loss-of-function and overexpression alleles on male gametophyte and sporophyte phenotypes as well as on auxin homoeostasis and metabolism revealed that PIN5 and PIN8 act antagonistically. This strongly suggests that PIN5 and PIN8 localized both at the same subcellular compartment (ER) can have distinct roles. In conclusion, this study identified auxin transporter PIN8 with a strong expression in a male gametophyte and revealed a role for auxin transport in regulating pollen development and function. Our results, including localization, auxin transport as well as genetic and physiological analyses, showed that, although both PIN8 and PIN5 auxin transporters are localized at the ER, they can have antagonistic roles in regulating gametophyte and sporophyte development, cellular auxin homoeostasis and metabolism. PIN5 has been proposed to transport auxin intracellularly from the cytoplasm into the ER, where enzymes involved in IAA metabolism are compartmentalized [6] , thus reducing the auxin availability for the PM-based auxin efflux [24] . It is unclear how PIN8 localized to the same intracellular compartment, namely ER, can act antagonistically but it suggests more complex functional interaction between PIN proteins than anticipated so far. A possible scenario would envision transient or more stable interaction of PIN5 and PIN8 negatively regulating each other transport capabilities. Notably, PIN8 activity in Arabidopsis is required only in male gametophyte. It is known that developing and germinating pollen has high levels of auxin [32] , but the auxin role there is unclear. Thus, it is possible that specifically during pollen development, the ER-localized PIN transporters regulate the release of auxin from the internal stores in the ER to drive auxin-mediated pollen tube elongation. The finding that some PIN proteins localize to the ER and other to the PM brings about an interesting question, namely, which of these functions and cellular localizations is ancestral and which physiological and developmental role did this ancestral PIN protein play. In the moss Physcomitrella , the most typical member of PIN clade localizes to ER, when expressed in BY-2 tobacco cells [24] . As in most ancestral land plants, the gametophyte generation is predominant, the male gametophytic PIN8 might represent a more ancestral form of auxin transporters that were at the ER involved in regulating subcellular auxin homoeostasis, before they acquired PM localization and new function in mediating auxin transport between cells for mediating development of higher plants. Nonetheless, also in higher plants, different ER-localized PIN proteins, including Arabidopsis PIN5, PIN8 and possibly also PIN6, have spatially and/or temporally distinct expression patterns [24] that can fine-tune the cellular free IAA levels optimal for plant growth and reproduction. Plant material and DNA constructs For all experiments, we used Arabidopsis thaliana ecotype Columbia (Col). Insertion mutant lines were pin5-5 (ref. 24 ), pin8-1 (Salk_107965) and pin8-2 (Salk_044651). Transgenic lines were DR5::GUS [29] , DR5rev::GFP [33] , RPS5A::GAL4 (ref. 34 ) and RPS5A >> PIN5-myc ( PIN5 OX ) [24] . pin5 pin8 double mutants and the PIN8OX PIN5OX double transgenic plants were generated through crossing pin5-5 with pin8-1 or crossing PIN8OX with PIN5OX . All SALK lines were obtained from the Nottingham Arabidopsis Stock Center. The 35S::PIN8-GFP ( PIN8 OX ) line was generated by transformation of the ecotype Columbia (Col) with the 35S::PIN8-GFP ( PIN8OX ) construct [24] . The LAT52::PIN8 line was generated via replacing the 35S promoter with the LAT52 promoter and transformed to the Colecotype. The primers used for cloning the LAT52 promoter are described in Supplementary Table S3 . Growth conditions Seeds were sterilized with chlorine gas and stratified at 4 °C for 3 days in the dark. Seedlings were grown vertically on half Murashige and Skoog (MS) medium supplemented with 1% sucrose and respective drugs. Drugs were purchased from Sigma-Aldrich. Plants were grown under the stable long-day (16 h light/8 h dark) or short-day (8 h light/16 h dark) conditions at 19 °C in growth chambers. Phenotype analyses and GUS (β-glucuronidase) staining Plates were scanned on a flat-bed scanner and hypocotyl lengths were measured with the ImageJ ( http://rsb.info.nih.gov/ij/ ) software. GUS staining was done as described [35] . Microscopy analysis The immunological analyses were done as previously described [36] . Details on antibodies and dilutions can be found in the later section. GFP samples were scanned without fixation. For confocal microscopy images, Zeiss LSM 510 or Olympus FV10 ASW confocal scanning microscopes were used. Pollen transmission assays We used the PIN3::PIN3-GFP line for the transmission wild-type controls. Pollen from the hetero PIN3::PIN3-GFP , hetero pin8-1 or hetero LAT52::PIN8 was used as a pollen donor, and crossed with Col female. Wild-type control–here is the hetero PIN3::PIN3-GFP line–showing around 50% transmission that was confirmed via antibiotic selection of the resulted seedlings. pin8-1 and LAT52::PIN8 transmission was assessed by PCR analysis or antibiotic selection of the resulted seedlings. Auxin measurements and transport assays Free IAA measurements and IAA metabolic profiling were done as described [24] . For protoplast transport assays, protoplasts prepared from loss-of-function mutant and overexpression lines were loaded under controlled conditions (loading is performed on ice in order to minimize transport processes with identical amounts of cells and radioactivity) leading to highly comparable loading of cells [22] . Loaded cells were then temperature shifted to 25 °C enabling catalysed auxin transport (of course both over the ER and PM membrane), and after defined time-points supernatants (containing effluxed radioactivity) were separated from cells by silicon oil centrifugation and quantified. For IAA conjugate quantification, ~10 mg of plant material was taken for analysis. The samples were processed as described [37] and quantified by ultra-high-performance liquid chromatography coupled to tandem mass detection. Auxin transport assays in ER-enriched microsomal fractions Arabidopsis plants grown in liquid culture were homogenized using razor blade in 5 ml of 0.5 M sucrose, 0.1 M KH 2 PO 4 (pH 6.65), 5 mM MgCl 2 and 1 mM dithiothreitol (freshly added). Membranes were separated following the procedure described by Muñoz et al . [38] , [39] . Briefly, the homogenate was filtered through miracloth (Calbiochem) and centrifuged at 3,000 g for 3 min. The supernatant was then layered on 5 ml of a 1.3 M sucrose cushion and centrifuged at 108,000 g for 90 min. The upper phase was removed without disturbing the interface fraction and sucrose layers of 1.1, 0.7 and 0.25 M were overlaid on the membrane pad. The discontinuous sucrose gradient was then centrifuged at 108,000 g for 90 min. The 1.1/1.3 M interface enriched in ER membranes was collected, diluted and centrifuged separately at 108,000 g for 50 min, the pellet was resuspended in 200 μl of 0.5 M sucrose, 0.1 M KH 2 PO 4 (pH 6.65) and 5 mM MgCl 2 and stored at −80 °C until use. ER-enriched membranes, obtained as described above, were used to perform [ 3 H]-IAA uptake assays, based in a filtration method previously described [39] . A total of 50 μg of protein from the ER-enriched membrane fraction were resuspended in a buffer containing 250 mM sucrose, 20 mM KCl, 25 mM Tris–HCl (pH 7). The reaction was initiated by adding 100 μl of 50 nM [ 3 H]-IAA (20 nCi), to reach 1 ml, final volume. Aliquots were taken at different times and filtered through 0.45-μm cellulose–ester filters (Millipore), previously treated with 250 mM sucrose, 20 mM KCl, 25 mM Tris–HCl (pH 7) and 1 mM IAA. The reaction was stopped by filtering and immediate wash using 5 ml of ice-cold 250 mM sucrose, 20 mM KCl, 25 mM Tris–HCl (pH 7) and 1 mM IAA. The filters were air-dried and the remaining radioactivity was measured in a liquid scintillation counter. The uptake of 3 H-IAA is reported in 'nmol of [ 3 H]-IAA/mg of protein'. Whole-mount immunolocalization and lifetime confocal microscopy Whole-mount immunological staining on 4-day-old seedlings was done in an Intavis robot. Antibodies were used at the following dilutions: rabbit anti-BIP2 (Hsc70), 1:200 (Stressgen Bioreagents); mouse anti-GFP, 1:600 (Roche); rabbit anti-myc, 1:600 (Sigma-Aldrich). Anti-rabbit and anti-mouse antibodies conjugated with Cy3 or fluorescein isothiocyanate (Dianova, Germany) were used at 1:600 dilutions. For ER-tracker dye labelling, PIN8::PIN8–GFP seedlings were mounted in water with a 1:1,000 dilution of ER-tracker dye (Invitrogen). Brefeldin A treatment for 2 h was performed by incubation of 4-day-old etiolated seedlings on solid MS medium supplemented with brefeldin A (50 μM), counterstaining of cell walls was achieved by mounting seedling roots in 10 μM propidium iodide. Quantitative PCR analysis RNA was extracted with the Plant RNeasy kit (Qiagen). Poly(dT) complementary DNA was prepared from flower total RNA. Superscript III reverse transcription (Invitrogen) and quantification were done on a LightCycler 480 apparatus (Roche Diagnostics) with the SYBR Green I Master kit (Roche Diagnostics), according to the manufacturer's instructions. All individual reactions were done in triplicate. Data were analysed as described before [40] . The primers used to quantify gene expression levels are provided in Supplementary Table S3 . Light and fluorescent microscopy For pollen phenotype observations, flowers from pin or Col-0 plants were collected to GUS buffer (0.1 M phosphate buffer, pH 7.0; 10 mM EDTA, pH 8.0; 0.1% triton X-100) supplemented with 100 ng ml −1 DAPI as described [41] . After 30-min incubation at room temperature in the dark, samples were analysed by bright-field and fluorescence microscopy with Nikon TE2000-E microscope (objective Nikon CFI Plan Fluor ELWD 10×/0.60, eyepiece Nikon CFI 10×/22, intermediate magnification ×1–×1.5; Nikon). Pollen germination in vitro Pollens were collected from flowers opened day (day 0) of Col and pin8-1 plants. Subsequently they were germinated on a germination medium on a microscope slide according to Boavida and McCormick [42] . Pollen germination medium was always prepared fresh from 0.5 M stock solutions of the main components (5 mM KCl, 0.01% H 3 BO 3 , 5 mM CaCl 2 , 1 mM MgSO 4 ) using autoclaved water. Sucrose (10%) was added and pH was adjusted to 7.5 with NaOH. Low-melting agarose (Amresco, Solon, OH) was added to final 1.5% concentration and melted in a microwave oven. Pollen grains from three flowers were spread on the surface of 250 μl agarose germination pads on microscope slides covered by polypropylene foil by inverting the flower with the help of tweezers and gently bringing it onto agarose surface. The whole flower was used as a 'brush' to spread pollen uniformly. The slides were incubated upside down in a moisture incubation chamber for 16 h in the dark at 22 °C and 100% humidity. The samples were examined by bright-field microscopy using Nikon TE2000-E microscope (objective Nikon CFI Plan UW 2×/0.06, eyepiece Nikon CFI 10×/22, intermediate magnification ×1–×1.5). The germinating pollen was defined as a pollen with a clearly visible pollen tube with length at least 1 diameter of pollen grain. The germination was carried out overnight (16 h). The percentage of germinated pollen was scored manually from captured image. From each microscope slide, five to six individual areas were taken. For NAA pollen germination test, 1 μM NAA was dissolved in the germination medium to 100 nM final concentration. How to cite this article: Ding, Z. et al . ER-localized auxin transporter PIN8 regulates auxin homoeostasis and male gametophyte development in Arabidopsis . Nat. Commun. 3:941 doi: 10.1038/ncomms1941 (2012).